Resolving the molecular mechanism of cadherin catch bond formation Classical cadherin Ca 2+ -dependent cell–cell adhesion proteins play key roles in embryogenesis and in maintaining tissue integrity. Cadherins mediate robust adhesion by binding in multiple conformations. One of these adhesive states, called an X-dimer, forms catch bonds that strengthen and become longer lived in the presence of mechanical force. Here we use single-molecule force-clamp spectroscopy with an atomic force microscope along with molecular dynamics and steered molecular dynamics simulations to resolve the molecular mechanisms underlying catch bond formation and the role of Ca 2+ ions in this process. Our data suggest that tensile force bends the cadherin extracellular region such that they form long-lived, force-induced hydrogen bonds that lock X-dimers into tighter contact. When Ca 2+ concentration is decreased, fewer de novo hydrogen bonds are formed and catch bond formation is eliminated. The establishment and maintenance of multicellular tissue structures, requires specific and robust adhesion of cells [1] . Proteins that play a key role in this process are the classical cadherin family of cell–cell adhesion proteins [2] . Robust cadherin adhesion is essential for maintaining the integrity of tissue such as the skin, blood vessels, cartilage and muscle that are exposed to continuous mechanical assault. Classical cadherin adhesion is also required for mediating cellular rearrangements during embryonic development. However, the mechanisms by which cadherins tune adhesion and withstand mechanical stress are not understood at the molecular level. Classical cadherins are Ca 2+ -dependent transmembrane proteins; adhesion is mediated by the binding of cadherin extracellular (EC) regions from opposing cells. This region is comprised of five EC domains that are arranged in tandem [3] , [4] , [5] . A network of Ca 2+ ions bound to the linker region between adjacent EC domains maintains the rigidity of the EC region [3] . Structural studies and single-molecule measurements show that cadherins from opposing cell surfaces bind in two distinct conformations [6] , [7] , [8] , [9] , [10] . The first conformation, called an X-dimer, is formed by extensive surface interactions via the two outer domains (EC1-2) of the cadherin EC region [6] , [9] . The second conformation, called a strand-swap dimer, is formed when the side chain of a conserved Tryptophan at position 2 (W2) is inserted into a pocket on the adhesive partner [7] , [11] . Recent single-molecule force measurements have shown that X-dimers form catch bonds that strengthen and increase their lifetimes when subjected to mechanical force [12] . Catch bonds presumably have important roles in cell migration and wound healing as they allow cells to grip strongly when pulled and to release in the absence of force [13] . However, the molecular mechanism that mediates X-dimer catch bond formation is not known. In contrast to X-dimers, strand-swap dimers form slip bonds that weaken when pulled [12] . However, the structural constraints that prevent strand-swap dimers from forming catch bonds are also unclear. Cadherin adhesion is compromised when Ca 2+ binding to the EC region is inhibited [14] ; for instance, mutations in the EC1-2 Ca 2+ -binding sites are observed in metastatic gastric cancers [15] , [16] . Although the role of Ca 2+ in strand-swap dimer formation is well understood [17] , the molecular mechanism by which Ca 2+ affects X-dimer adhesion is unknown. In this paper, we resolve the molecular interactions by which X-dimers of E-cadherin, a prototypical classical cadherin, form catch bonds. We also identify the molecular mechanisms by which Ca 2+ ions regulate this process. We first use molecular dynamics (MD) and steered MD (SMD) simulations to identify both the amino acids involved in catch bond formation and to predict the effect of Ca 2+ ions on X-dimer catch bonds. We then experimentally test these predictions at the single-molecule level using force-clamp spectroscopy measurements with an atomic force microscope (AFM). Our results show that tensile force orients the cadherins such that they form several de novo hydrogen bonds that are capable of withstanding force; a majority of these bonds are formed by amino acids located on the N-terminal β-strands on the EC1 domain. Since these β-strands are exchanged during the process of strand-swapping [7] , strand-swap dimers do not form force-induced H-bonds. When the cadherin EC region is made more flexible by reducing the Ca 2+ concentration, fewer force-induced bonds are formed; consequently, catch bonds are eliminated. Our experimental data can be described by a sliding–rebinding model where application of a tensile force rearranges the cadherin ectodomains and results in the formation of force-induced interactions [18] , [19] . X-dimers become disordered as Ca 2+ concentration decreases We used MD simulations to examine the role of Ca 2+ ions in maintaining the rigidity of E-cadherin X-dimers. Since X-ray crystallography [6] and single-molecule fluorescence resonance energy transfer measurements [9] have shown that cadherins can be trapped in an X-dimer conformation by mutating the swapped amino-acid W2 to alanine (W2A), the crystal structure of the EC1-2 domains of E-cadherin W2A mutants (pdb: 3LNH) [6] were used in the simulations. Different solution Ca 2+ concentrations were simulated by varying the number of Ca 2+ ions bound to the linker between the EC1 and EC2 domains. Since each EC1-2 linker binds cooperatively to three Ca 2+ ions [20] , [21] , [22] , [23] , physiological Ca 2+ concentrations were simulated by binding six Ca 2+ ions to the X-dimer. Lower solution Ca 2+ concentrations were simulated by eliminating one, two or all three Ca 2+ ions from each linker in the X-dimer. The Ca 2+ ions bound to the X-dimer are labelled CA1, CA2 and CA3, and illustrated in Supplementary Fig. 1 ; Ca 2+ ions that interacted with fewer number of acidic amino acids were preferentially removed (in order of increasing number of negatively charged neighbours: CA1<CA2<CA3; Supplementary Fig. 1 ). In order to obtain reliable statistics on X-dimer hydrogen bonds (H-bonds) under force-free conditions, three MD simulations for each condition (6 Ca 2+ , 4 Ca 2+ , 2 Ca 2+ and 0 Ca 2+ ) were carried out using GROMACS with a GROMOS all-atom force field [24] , [25] . Before equilibration, the X-dimers were solvated in a water box and neutralized with Na + counter-ions, and energy was minimized. MD simulations for 10 ns (X-dimers bound to 6 Ca 2+ ions), 16 ns (X-dimers bound to 4 Ca 2+ ions and 2 Ca 2+ ions) and 30 ns (X-dimers without any Ca 2+ ions) were then performed in 2 fs integration time steps ( Fig. 1 ). 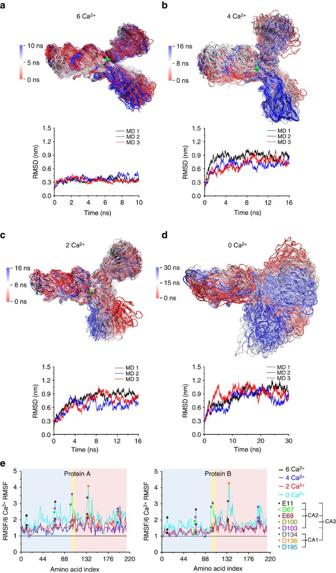Figure 1: X-dimers become disordered as Ca2+concentration is decreased. The rigidity of the EC1-2 domains of X-dimers bound to either 6 Ca2+, 4 Ca2+, 2 Ca2+or 0 Ca2+ions were predicted using molecular dynamics (MD) simulations; three simulations were carried out for each condition. For better visibility, only 50 frames of one simulation for each condition are displayed and the EC1 domain of protein B is constrained to the initial structure. Frames at the start of simulation are in red, whereas frames at the end are in blue. Ca2+ions are displayed as green spheres. Root mean squared deviation (RMSD) listed below correspond to the average RMSD following equilibration, for all three simulations. X-dimers bound to (a) 6 Ca2+ions (10 ns MD simulations), RMSD=3.6 Å; (b) 4 Ca2+ions (16 ns MD simulations), RMSD=7.9 Å; (c) 2 Ca2+ions (16 ns MD simulations), RMSD=7.7 Å; and (d) no Ca2+ions (30 ns MD simulations), RMSD=9.3 Å. (e) The average root mean square fluctuation (RMSF) in all three MD simulations were normalized by the average RMSFs of the X-dimer bound to 6 Ca2+ions. Lightly shaded regions distinguish the residues in the EC1 domain (blue), linker (yellow) and EC2 domain (red). Figure 1: X-dimers become disordered as Ca 2+ concentration is decreased. The rigidity of the EC1-2 domains of X-dimers bound to either 6 Ca 2+ , 4 Ca 2+ , 2 Ca 2+ or 0 Ca 2+ ions were predicted using molecular dynamics (MD) simulations; three simulations were carried out for each condition. For better visibility, only 50 frames of one simulation for each condition are displayed and the EC1 domain of protein B is constrained to the initial structure. Frames at the start of simulation are in red, whereas frames at the end are in blue. Ca 2+ ions are displayed as green spheres. Root mean squared deviation (RMSD) listed below correspond to the average RMSD following equilibration, for all three simulations. X-dimers bound to ( a ) 6 Ca 2+ ions (10 ns MD simulations), RMSD=3.6 Å; ( b ) 4 Ca 2+ ions (16 ns MD simulations), RMSD=7.9 Å; ( c ) 2 Ca 2+ ions (16 ns MD simulations), RMSD=7.7 Å; and ( d ) no Ca 2+ ions (30 ns MD simulations), RMSD=9.3 Å. ( e ) The average root mean square fluctuation (RMSF) in all three MD simulations were normalized by the average RMSFs of the X-dimer bound to 6 Ca 2+ ions. Lightly shaded regions distinguish the residues in the EC1 domain (blue), linker (yellow) and EC2 domain (red). Full size image Although the stability of X-dimers under saturating and Ca 2+ -free conditions have been previously studied [26] , the dynamics of X-dimers bound to different numbers of Ca 2+ ions has not been examined. In agreement with previous MD simulations [26] , [27] , our results indicate that X-dimers become more flexible as the Ca 2+ concentration is decreased. X-dimers bound to 6 Ca 2+ ions displayed the least motion in all three MD simulations; they rapidly equilibrated within ~270 ps and the root mean square deviation (RMSD) remained fairly constant throughout the rest of the simulation with an average value of 3.6 Å ( Fig. 1a ). On the other hand, X-dimers bound to 4 Ca 2+ ions ( Fig. 1b ) and 2 Ca 2+ ions ( Fig. 1c ) equilibrated more slowly over ~3 and ~5 ns, respectively. Following equilibration, these X-dimers showed comparable motion with average RMSDs of 7.9 and 7.7 Å, respectively ( Fig 1b,c ). In the absence of Ca 2+ , the cadherin ectodomain became very flexible and required an average of ~9 ns to equilibrate; the average RMSD, following equilibration increased to 9.3 Å ( Fig. 1d ). Previous studies suggest that cadherins become more disordered in the absence of Ca 2+ due to repulsion between negatively charged amino acids in the Ca 2+ -binding sites [26] , [27] . To confirm this, we calculated the root mean square fluctuation (RMSF) of every amino acid in the X-dimer (the opposing binding partners in the X-dimer are henceforth referred to as proteins ‘A’ and ‘B’); the calculated RMSF normalized by the corresponding value in the 6 Ca 2+ ion simulation is plotted in Fig. 1e . Our data show that the RMSFs were 2–4 times higher in the absence of Ca 2+ compared with X-dimers saturated with 6 Ca 2+ ions ( Fig. 1e ). In both proteins A and B, amino acids in the CA1-binding site (D134, D136 and D195) had the largest normalized RMSF, whereas the normalized RMSFs of CA2 and CA3 coordinating residues were comparable in magnitude ( Fig. 1e ). Force-induced hydrogen bond formation is Ca 2+ dependent Based on their higher RMSDs, we predicted that X-dimers bound to fewer than 6 Ca 2+ ions will be unable to lock together and form catch bonds when pulled. To test this, we used explicit solvent SMD to monitor the formation of force-dependent, de novo intermolecular interactions when a tensile force was applied to X-dimers bound to different numbers of Ca 2+ ions. Although SMD simulations have previously been used to study the force-induced dissociation of strand-swap dimers [28] , the force-induced unbinding of X-dimers has not been examined. X-dimer structures from the last frame of the MD simulations were used as the starting point in the SMD simulations. Two constant velocity SMD simulations, one with pulling rate of 2 nm ns −1 (referred as fast SMD) and another at a velocity of 0.4 nm ns −1 (henceforth labelled as slow SMD) were performed on X-dimers bound to 6, 4, 2 and 0 Ca 2+ ions. The X-dimers were pulled by applying a harmonic potential between the C terminus of each cadherin; while the C terminus of protein A served as the reference, the C terminus of protein B was designated as the pulling group. Simulations were terminated when the cadherins dissociated ( Supplementary Videos 1–8 ). SMD simulations show that catch bond formation is mechanically regulated by the flexibility of the ectodomain. When X-dimers are bound to 6 Ca 2+ ions, their linkers become rigid. Consequently, the pulling force flexes each ectodomain and slides opposing EC1 domains such that previously well separated, yet complementary, amino acids are brought into registry resulting in the formation of de novo , force-induced H-bonds ( Figs 2a and 3a–e , and Supplementary Fig. 2a ). However, when X-dimers are not saturated with Ca 2+ ions, the linkers become more flexible and bend independent of the EC1 domains. As a result, the number of force-induced H-bonds are reduced when the X-dimers associate with 4, 2, or 0 Ca 2+ ions ( Figs 2b–d and 3f–k , and Supplementary Figs 2b–d and 3a–c ). 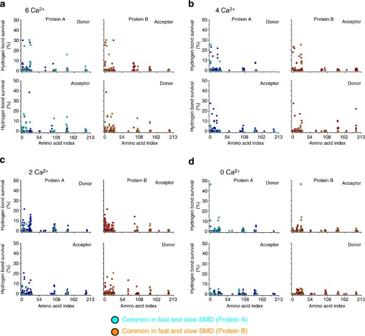Figure 2: Lifetimes of force-induced H-bonds increase with number of Ca2+ions bound to the X-dimer. Survival probability (the fraction of total simulation time for which an H-bond survives) is plotted for each donor and acceptor amino acid in the X-dimer. The four plots in each panel correspond to H-bonds formed between donors on protein A (upper left) and corresponding acceptors on protein B (upper right), and H-bonds formed between acceptors on protein A (lower left) and corresponding donors on protein B (lower right). Blue and cyan dots correspond to donors and acceptors on protein A, whereas red and orange dots refer to amino acids in protein B. Cyan and orange dots correspond to hydrogen bonds that are measured in both slow and fast SMD simulations under the same Ca2+conditions. Donor–acceptor pairs in (a) 6 Ca2+(b) 4 Ca2+(c) 2 Ca2+and (d) 0 Ca2+ions shows that X-dimers bound to 6 Ca2+have higher number of long-lived, force-induced H-bonds. Figure 2: Lifetimes of force-induced H-bonds increase with number of Ca 2+ ions bound to the X-dimer. Survival probability (the fraction of total simulation time for which an H-bond survives) is plotted for each donor and acceptor amino acid in the X-dimer. The four plots in each panel correspond to H-bonds formed between donors on protein A (upper left) and corresponding acceptors on protein B (upper right), and H-bonds formed between acceptors on protein A (lower left) and corresponding donors on protein B (lower right). Blue and cyan dots correspond to donors and acceptors on protein A, whereas red and orange dots refer to amino acids in protein B. Cyan and orange dots correspond to hydrogen bonds that are measured in both slow and fast SMD simulations under the same Ca 2+ conditions. Donor–acceptor pairs in ( a ) 6 Ca 2+ ( b ) 4 Ca 2+ ( c ) 2 Ca 2+ and ( d ) 0 Ca 2+ ions shows that X-dimers bound to 6 Ca 2+ have higher number of long-lived, force-induced H-bonds. 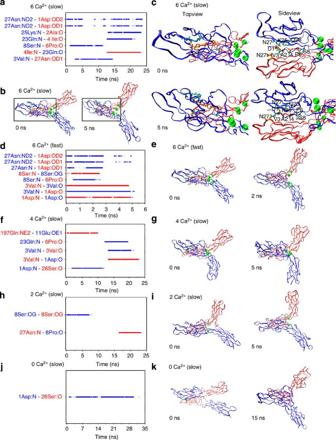Figure 3: Long-lived, force-induced H-bonds are formed by the sliding and rebinding of opposing ectodomains under physiological Ca2+conditions. The number of thesede novoH-bonds decreases as the number of Ca2+ions bound to the X-dimer is reduced. (a) In slow steered molecular dynamics (SMD) simulations, X-dimers bound to 6 Ca2+ions form seven long-lived H-bonds. (b) Tensile force flexes the cadherin ectodomain (0 and 5 ns snapshots from slow SMD simulation); and (c) rearranges opposing EC1 domains such that H-bond donor and acceptor amino acids are brought into registry. Top and side views of boxed regions inbbefore (0 ns) and after (5 ns) EC1 rearrangement are shown. (d) In fast SMD simulations, X-dimers bound to 6 Ca2+ions form eight long-lived,de novoH-bonds by (e) flexing of the EC region (snapshots at 0 ns and 2 ns). (f) Slow SMD simulations show that X-dimers bound to 4 Ca2+ions form five force-induced bonds, (g) corresponding snapshots at 0 and 5 ns. (h) Similarly, X-dimers bound to 2 Ca2+ions form two long-livedde novoH-bonds, (i) corresponding snapshots at 0 and 5 ns. (j) Finally, slow SMD simulations show that in the absence of Ca2+ions, X-dimers form one force-induced H-bond, (k) snapshots at 0 ns and during flexing at 15 ns. Ina,d,f,handj, every frame where an H-bond exists is denoted by a point; blue points correspond to H-bonds formed by donors on protein A, whereas red points correspond to bonds formed by donors on protein B. Inb,c,e,g,iandk, Protein A is in blue and Protein B is in red. Full size image Figure 3: Long-lived, force-induced H-bonds are formed by the sliding and rebinding of opposing ectodomains under physiological Ca 2+ conditions. The number of these de novo H-bonds decreases as the number of Ca 2+ ions bound to the X-dimer is reduced. ( a ) In slow steered molecular dynamics (SMD) simulations, X-dimers bound to 6 Ca 2+ ions form seven long-lived H-bonds. ( b ) Tensile force flexes the cadherin ectodomain (0 and 5 ns snapshots from slow SMD simulation); and ( c ) rearranges opposing EC1 domains such that H-bond donor and acceptor amino acids are brought into registry. Top and side views of boxed regions in b before (0 ns) and after (5 ns) EC1 rearrangement are shown. ( d ) In fast SMD simulations, X-dimers bound to 6 Ca 2+ ions form eight long-lived, de novo H-bonds by ( e ) flexing of the EC region (snapshots at 0 ns and 2 ns). ( f ) Slow SMD simulations show that X-dimers bound to 4 Ca 2+ ions form five force-induced bonds, ( g ) corresponding snapshots at 0 and 5 ns. ( h ) Similarly, X-dimers bound to 2 Ca 2+ ions form two long-lived de novo H-bonds, ( i ) corresponding snapshots at 0 and 5 ns. ( j ) Finally, slow SMD simulations show that in the absence of Ca 2+ ions, X-dimers form one force-induced H-bond, ( k ) snapshots at 0 ns and during flexing at 15 ns. In a , d , f , h and j , every frame where an H-bond exists is denoted by a point; blue points correspond to H-bonds formed by donors on protein A, whereas red points correspond to bonds formed by donors on protein B. In b , c , e , g , i and k , Protein A is in blue and Protein B is in red. Full size image When the X-dimers are pulled in the SMD simulations, flexing of proteins A and B ( Fig. 3b,e,g,i,k , and Supplementary Fig. 3d–3f ) reduces the angle between the long axis of their EC1 and EC2 domains from the original angle of 163° measured in the crystal structure ( Supplementary Fig. 4 ). For X-dimers with stiff linkers, that are bound to 6 Ca 2+ ions, the EC1–EC2 angle on both proteins A and B, when the proteins are completely flexed, reduces by 31° and 30° (slow SMD) and 47° and 40° (fast SMD), respectively ( Supplementary Fig. 4a ). In contrast, when the linkers are not saturated with Ca 2+ , bending is increased; consequently the EC1–EC2 angle is reduced by a larger amount. For example, when X-dimers are bound to 4 Ca 2+ ions, the EC1–EC2 angle for the slow SMD and the fast SMD decreases by 80° and 65° (protein A) and 62° and 69° (protein B), respectively ( Supplementary Fig. 4b ). Similarly, when X-dimers are associated with 2 Ca 2+ ions, the angle between the EC1 and EC2 domains, on proteins A and B by decrease by 55° and 75° (slow SMD) and 66° and 59° (fast SMD), respectively ( Supplementary Fig. 4c ). Finally, this angle reduces by 68° and 90° (slow SMD) and 83° and 67° (fast SMD) for X-dimers in the absence of Ca 2+ ions ( Supplementary Fig. 4d ). Since the MD and SMD simulations define H-bond formation by the satisfaction of certain distance (H-bond acceptor–donor distance <3.5 Å) and angle (acceptor-donor-hydrogen angle <30°) constraints, dynamic motion of opposing cadherins result in the identification of numerous H-bonds, most of which are very short-lived (<0.5% of the duration of the simulation). To distinguish between these transient H-bonds and longer-lived interactions in the MD simulations, we established an empirical criterion that H-bonds between proteins A and B, which exist for >40% of the equilibrated portion of the simulations, were force-free, permanent interactions ( Supplementary Fig. 5 ). In the SMD simulations, H-bonds were classified as force-induced interactions if they were not permanent interactions in the force-free MD simulations ( Fig. 2 ). These force-induced H-bonds were further classified as long-lived interactions if they existed for >20% of the duration of the SMD simulation ( Fig. 3 and Supplementary Fig. 3a–c ). It should be noted that while the 40 and 20% survival probability thresholds for classifying H-bonds as force-free and force-induced interactions were empirically established, altering these criteria only changed the absolute number of H-bonds, the trends measured across the different Ca 2+ conditions remain unaltered. When X-dimers bound to 6 Ca 2+ ions were pulled, the numbers of long-lived, force-induced H-bonds were higher for both the fast and slow SMD simulations compared with all other Ca 2+ conditions ( Fig. 3 ). For X-dimers bound to 6 Ca 2+ , the amino acids that form force-induced H-bonds in the slow and fast SMD simulations were located either at the apex of EC1 domains (Q23, K25 and N27) or at the N-terminal β-strand (D1, A2, V3, I4, P6 and S8) ( Fig. 3c ). As the ectodomains flexed in the slow SMD simulation ( Fig. 3b ), N27, K25, Q23, S8 and V3 on Protein A slid into alignment with D1, A2, I4, P6 and N27 on Protein B and formed seven de novo H-bonds ( Fig. 3a,c ). Similarly, eight force-induced H-bonds were formed in the fast SMD by the binding of N27, S8, V3 and D1 on Protein A with D1, S8, P6 and V3 on Protein B ( Fig. 3d ). Three of these long-lived, force-induced H-bonds (8Ser:N-6Pro:O, 27Asn:ND2-1Asp:OD2 and 27Asn:ND2-1Asp:OD1), were identical in both the slow and fast SMD simulations. In contrast, when each EC1-2 linker was bound to <6 Ca 2+ ions, the number of long-lived, force-induced hydrogen bonds decreased. In the case of X-dimers bound to 4 Ca 2+ ions, five de novo interactions were measured in both slow and fast SMD simulations ( Fig. 3f and Supplementary Fig. 3a ). On the other hand, X-dimers associated with 2 Ca 2+ ions formed two (slow) ( Fig. 3h ) and six (fast) ( Supplementary Fig. 3b ) force-induced H-bonds. Finally, in Ca 2+ -free conditions, X-dimers formed only one and four de novo H-bonds in the slow and fast SMD simulations, respectively ( Fig. 3j and Supplementary Fig. 3c ). The hydrophobic and hydrophilic accessible surface area was not lower when X-dimers were bound to 6 Ca 2+ ions, suggesting that no force-induced hydrophobic or van der Waals interactions are formed at saturating Ca 2+ concentrations ( Supplementary Fig. 6 ). Taken together, our simulations suggest that the higher number of long-lived, force-induced H-bonds formed at physiological Ca 2+ concentrations are responsible for X-dimer catch bonds. X-dimers form catch bonds at Ca 2+ concentrations ⩾ 1 mM We experimentally tested the predicted effect of Ca 2+ concentration on X-dimer catch bonds using single-molecule AFM force-clamp spectroscopy ( Fig. 4 ) [13] . W2A mutants of the complete E-cadherin ectodomain were engineered to trap the protein in an X-dimer conformation [6] . The cadherins were site specifically biotinylated at their C terminus to a 15 amino-acid AviTag sequence, and immobilized on an AFM tip and substrate using a Polyethylene glycol (PEG) tether ( Fig. 4a ) [9] , [12] , [29] . The tip and substrate were brought into contact to allow opposing W2A cadherins to form X-dimers. The AFM tip was then withdrawn from the substrate and clamped at a pre-determined force. 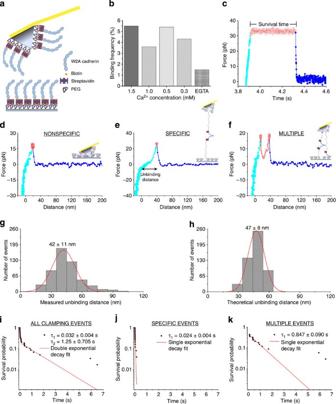Figure 4: Single-molecule force-clamp experiments on cadherin X-dimers. (a) Biotinylated W2A cadherins were immobilized on AFM tips and substrates functionalized with polyethylene glycol (PEG) linkers, some of which were decorated with streptavidin molecules. (b) In the presence of 1.5 and 1 mM Ca2+, and 500 and 300 μM Ca2+, the binding frequency was ~4%. In contrast, <2% binding events were measured when Ca2+was chelated using EGTA. (c) Typical data obtained in an AFM force-clamp experiment. To rupture X-dimers, the tip was separated from the surface (cyan) and then clamped at a constant force (red). When the X-dimer ruptured, the AFM cantilever recoiled back to its equilibrium position (blue). Survival time at the clamping force was determined from the period of time that the X-dimer persisted. In order to distinguish single-molecule events from unresolved multiple binding and nonspecific adhesion, the force-clamp data was converted to the corresponding force versus distance trace and stretching of the PEG tether was monitored (cyan, red and blue circles ind,eandfcorrespond to the tip-surface separation, force-clamp and recoil regions described inc). (d) Nonspecific unbinding. (e) Specific X-dimer unbinding. (f) Multiple unbinding events. For specific X-dimer unbinding events, the unbinding distances that were (g) measured and (h) calculated using a Freely Jointed Chain model for PEG extension in water quantitatively agree. (i) X-dimer bond survival probability when specific binding is not filtered out from nonspecific and multiple adhesion events decays as the sum of two exponentials. (j) Survival probabilities for specific single-molecule unbinding events inidecay as the short lifetime single exponential. (k) Survival probabilities for multiple unbinding events inidecay as the long lifetime single exponential. Figure 4: Single-molecule force-clamp experiments on cadherin X-dimers. ( a ) Biotinylated W2A cadherins were immobilized on AFM tips and substrates functionalized with polyethylene glycol (PEG) linkers, some of which were decorated with streptavidin molecules. ( b ) In the presence of 1.5 and 1 mM Ca 2+ , and 500 and 300 μM Ca 2+ , the binding frequency was ~4%. In contrast, <2% binding events were measured when Ca 2+ was chelated using EGTA. ( c ) Typical data obtained in an AFM force-clamp experiment. To rupture X-dimers, the tip was separated from the surface (cyan) and then clamped at a constant force (red). When the X-dimer ruptured, the AFM cantilever recoiled back to its equilibrium position (blue). Survival time at the clamping force was determined from the period of time that the X-dimer persisted. In order to distinguish single-molecule events from unresolved multiple binding and nonspecific adhesion, the force-clamp data was converted to the corresponding force versus distance trace and stretching of the PEG tether was monitored (cyan, red and blue circles in d , e and f correspond to the tip-surface separation, force-clamp and recoil regions described in c ). ( d ) Nonspecific unbinding. ( e ) Specific X-dimer unbinding. ( f ) Multiple unbinding events. For specific X-dimer unbinding events, the unbinding distances that were ( g ) measured and ( h ) calculated using a Freely Jointed Chain model for PEG extension in water quantitatively agree. ( i ) X-dimer bond survival probability when specific binding is not filtered out from nonspecific and multiple adhesion events decays as the sum of two exponentials. ( j ) Survival probabilities for specific single-molecule unbinding events in i decay as the short lifetime single exponential. ( k ) Survival probabilities for multiple unbinding events in i decay as the long lifetime single exponential. Full size image Binding of W2A cadherins were highly specific and Ca 2+ dependent; while a binding probability of ~4% was measured at [Ca 2+ ] ⩾ 300 μM, <2% binding events were measured with the same surface when free Ca 2+ was chelated from solution using EGTA ( Fig. 4b ). Cadherin-binding frequency was adjusted to ~4% by controlling the cadherin density on the tip and substrate ( Fig. 4b ); Poisson statistics predicts that under these conditions, >97% of measured events occur because of the rupture of single X-dimers. Single-molecule fluorescence microscopy experiments have previously shown that under similar experimental conditions, a majority of the measured unbinding events occur because of rupture of single trans -dimers [29] . Approximately 1,000–2,000 single-molecule measurements were carried out at five different clamping forces. The lifetime of each event was measured from the persistence time of the X-dimer interaction ( Fig. 4c ). Bond lifetime at each clamping force was determined from single-exponential decay fits to the bond survival probability [12] , [30] . As reported elsewhere [12] , [31] , [32] , [33] , cadherin bond survival probabilities decayed as the sum of two exponentials that correspond to the existence of two bound states ( Fig. 4i ). Previously, using control experiments, we had indirectly shown that the adhesive state with higher probability occurs owing to X-dimer unbinding, whereas the low probability state arises from nonspecific adhesion [12] . In order to directly identify single-molecule unbinding events and eliminate the unresolved unbinding of multiple molecules and nonspecific adhesion, force-clamp measurements were converted to the corresponding force versus distance traces and stretching of the PEG tether that anchor X-dimers to the substrate/AFM tip was monitored ( Fig 4d–f ). The stretching of PEG served as a molecular fingerprint for single-molecule unbinding, as its extension under load has been extensively characterized [34] , [35] . PEG stretching was not observed in the case of nonspecific adhesion ( Fig. 4d ). Specific binding was identified by single-stretching events ( Fig. 4e ), whereas the unbinding of multiple molecules resulted in the extension of multiple polymers ( Fig. 4f ). For every unbinding event, we measured the unbinding distance and compared it with the corresponding distance calculated using a freely jointed chain model for PEG stretching in water (see Methods section) [35] . For specific interactions, an excellent agreement between the theoretical predictions and experimental measurements was observed; the measured and predicted unbinding lengths were normally distributed with mean±s.d. values of 42±11 and 47±8 nm, respectively ( Fig. 4g,h ). Filtering specific single-molecule unbinding ( Fig. 4j ) from the contaminating nonspecific and multiple adhesion events resulted in the elimination of a majority of events that had long lifetimes ( Fig. 4i,k ). Consequently, the filtered bond survival probabilities decayed as a single exponential ( Fig. 4j and Fig. 5 , inset). 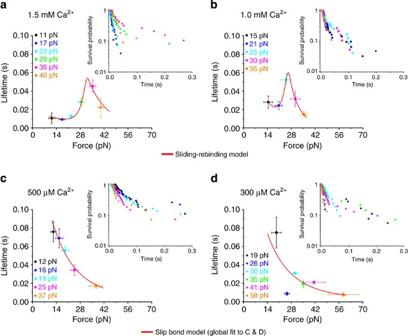Figure 5: At Ca2+concentrations⩾1 mM, X-dimers form catch bonds, whereas at lower Ca2+concentrations they form slip bonds. Bond lifetimes at the different clamping forces were determined from single-exponential decay fits to the corresponding bond survival probabilities (insets); a few long lifetime events have been eliminated for clarity. Survival probabilities and lifetimes are colour coded according to the corresponding clamping force. Error bars in lifetime correspond to s.e., whereas error bars in force correspond to s.d. In (a) 1.5 mM Ca2+and (b) 1 mM Ca2+, the X-dimers form catch-slip bonds that were fitted to a sliding–rebinding model (red). At lower Ca2+concentrations of (c) 500 μM and (d) 300 μM, the X-dimers form slip bonds that were globally fit to a slip bond model (red). Figure 5: At Ca 2+ concentrations ⩾ 1 mM, X-dimers form catch bonds, whereas at lower Ca 2+ concentrations they form slip bonds. Bond lifetimes at the different clamping forces were determined from single-exponential decay fits to the corresponding bond survival probabilities (insets); a few long lifetime events have been eliminated for clarity. Survival probabilities and lifetimes are colour coded according to the corresponding clamping force. Error bars in lifetime correspond to s.e., whereas error bars in force correspond to s.d. In ( a ) 1.5 mM Ca 2+ and ( b ) 1 mM Ca 2+ , the X-dimers form catch-slip bonds that were fitted to a sliding–rebinding model (red). At lower Ca 2+ concentrations of ( c ) 500 μM and ( d ) 300 μM, the X-dimers form slip bonds that were globally fit to a slip bond model (red). Full size image To confirm that the measured lifetimes were not a result of failure of the streptavidin–biotin interactions that were used to immobilize the cadherins on the AFM tip and surface, we measured the force-dependent lifetimes of the bonds formed between single biotinylated PEG tethers functionalized on an AFM tip and streptavidin immobilized on the substrate ( Supplementary Fig. 7 ). The experiments showed that streptavidin and biotin form slip bonds; the lifetime of this interaction, at all clamping forces, was more than an order of magnitude larger than the X-dimer lifetimes measured in our experiments ( Supplementary Fig. 7 ). We measured X-dimer catch bond formation at four different free Ca 2+ concentrations: 1.5 and 1 mM, and 500 and 300 μM, respectively ( Fig. 5 ). In 1.5 mM Ca 2+ ( Fig. 5a ) and 1 mM Ca 2+ ( Fig. 5b ), where each EC1-2 linker is expected to bind to 3 Ca 2+ ions, the X-dimers formed catch-slip bonds. The bond lifetimes initially increased with force, indicative of a catch bond. After reaching a maximum at a critical force of ~27–32 pN, the lifetimes decreased with force, indicating slip bond behaviour. Previously, we have shown that X-dimers form similar catch-slip bonds at a Ca 2+ concentration of 2.5 mM [12] . Simulations of X-dimers bound to 6 Ca 2+ ions show that tensile force results in the rearrangement of opposing EC1 domains followed by the formation of long-lived, force-induced interactions. We therefore fit the experimental catch-slip bond data to a sliding–rebinding model that predicts that catch bonds are formed when an external force induces a receptor and ligand to slide relative to each other and rebind in a second conformation, with new interactions. Fits to this model ( Supplementary Table 1 ) showed an excellent quantitative agreement with the experimental data measured at 1.5 mM Ca 2+ ( Fig. 5a ) and 1.0 mM Ca 2+ ( Fig. 5b ). In contrast, when the Ca 2+ concentration was decreased such that each EC1-2 linker was bound to either 2 Ca 2+ ions or 1 Ca 2+ ion, catch bond formation was abolished ( Fig. 5c,d ). At Ca 2+ concentrations of 500 μM ( Fig. 5c ) and 300 μM ( Fig. 5d ), the X-dimers formed slip bonds; their bond lifetimes decreased with increasing tensile force. We globally fit this data to a previously described model for slip bond formation to obtain parameters that best fit all data sets [36] . The fits yielded an intrinsic bond lifetime in the absence of force of 0.21 s ( Supplementary Table 2 ). In summary, we used computer simulations and single-molecule force measurements to show that tensile force flexes X-dimers such that they slide into registry and form long-lived, force-induced hydrogen bonds that lock them into tighter contact. These force-induced interactions, which are not observed under force-free conditions, are formed at Ca 2+ concentrations ⩾ 1 mM when each EC1-2 linker is saturated with 3 Ca 2+ ions. Removing one Ca 2+ (CA1) from the EC1-2 linker eliminates this force-induced H-bond formation. It has been reported that mutation of a conserved A144 (also numbered A298 when the signal and pro-peptide are included), next to one of the CA1 coordinating residues in the EC1-2 linker, occurs in diffuse gastric cadherin [15] , [16] . It is a possibility that X-dimer catch bond formation is hindered in this metastatic cancer cell line. Similar to E-cadherins, the stiffness and molecular strength of non-classical cadherin-23, which is an essential component of the hair-cell tip link, is mediated by the binding of Ca 2+ ions [37] . Mutations of Ca 2+ -binding residues, which occur in some forms of deafness, render tip links prone to mechanical failure [37] . Previous studies [12] also show that unlike X-dimers, cadherin strand-swap dimers do not form catch bonds. Our SMD simulations suggest that this is because a majority of the acceptors involved in these force-induced H-bonds are located in or around the N-terminal β-strands on the EC1 domains. In strand-swap dimers, the N-terminal β-strands are exchanged between opposing EC1 domains [7] , and consequently are in an orientation that prevents the formation of force-induced H-bonds. In agreement with previous studies that used Amber [26] and CHARMM [27] force fields, our study using a GROMOS all-atom force field also shows that saturating the EC linkers with Ca 2+ ions is essential to maintain the rigidity of the W2A cadherin ectodomain. Based on the increased flexibility of X-dimers bound to fewer than 3 Ca 2+ ions per linker, we hypothesized that X-dimers that are not saturated with Ca 2+ ions will be unable to form force-induced bonds because of their inability to slide into registry when flexed. We confirmed this hypothesis using explicit solvent SMD simulations carried out at both slow and fast pulling velocities. Although even the slow SMD simulations have loading rates that are several orders of magnitude larger than the experimental force ramp rates, recent measurements show an excellent, quantitative agreement between high-speed AFM force spectroscopy experiments and SMD simulations [38] . Our SMD simulations show that while X-dimers bound to 6 Ca 2+ ions form 7–8 long-lived, force-induced H-bonds, removing even one Ca 2+ (CA1) from the EC1-2 linker reduces the number of these de novo H-bonds. The formation of 7–8 de novo H-bonds are more than sufficient to prolong the lifetime of X-dimers to the maximum of ~0.06 s measured in our experiments ( Fig. 5a,b ). AFM force spectroscopy and electron-tunnelling experiments show that just four H-bonds are sufficient to bind a single nucleotide to synthetic recognition agents for ~4 s (ref. 39 ). Similarly, AFM force spectroscopy experiments show that the lifetime of single base-pairs formed via either 2 or 3 H-bonds is ~2 and 4 s, respectively [40] . Furthermore, these experiments show that H-bonds exhibit lifetimes larger than 0.1 s even in the presence of 40–60 pN load [40] . Affinity measurements indicate that the binding of Ca 2+ ions to the cadherin ectodomain have K D ’s ranging anywhere between 20 μM and 460 μM (refs 20 , 21 , 23 , 37 , 41 , 42 ). Furthermore, measurements suggest that the binding of Ca 2+ to the EC linkers has a positive cooperativity; various Hill coefficients ranging up to 3.7 have been reported in the literature [20] , [21] , [22] , [23] , [37] . Owing to wide variations in the measured affinity of the ectodomain for Ca 2+ ions, we tested the force-dependent binding kinetics of X-dimers at Ca 2+ concentrations ranging from 1.5 mM to 300 μM; studies show that the cadherin ectodomain stiffens and adopt an extended trans-dimer conformation at solution Ca 2+ concentrations of 1 mM (refs 14 , 22 ). As suggested by the SMD simulations, X-dimers formed catch-slip bonds in 1.5 and 1 mM Ca 2+ where the ectodomains are stiff and each EC1-2 linker binds to 3 Ca 2+ ions. However, at Ca 2+ concentrations of 500 and 300 μM, the X-dimers formed slip bonds. Several alternate models have been proposed to describe receptor-ligand catch bond formation [13] . These include energy landscapes with one bound state and two unbinding pathways [43] ; an energy landscape with two bound states, one of which is preferentially stabilized by force [44] , [45] ; bond dissociation along a multidimensional landscape where the direction of the tensile force and the reaction coordinate are misaligned [46] , [47] , [48] ; a free-energy landscape with dynamic disorder that thermally fluctuates with time [49] , [50] ; and allosteric deformation models where external force changes the structure of the receptor either directly at the ligand-binding site [51] or at a distal location that ultimately propagates the deformation to the binding pocket [52] , [53] , [54] , [55] . Our simulations suggest that X-dimers form catch bonds via a sliding–rebinding mechanism where a pulling force flexes the ectodomain and slides opposing EC1 domains resulting in the formation of de novo , force-induced H-bonds. The experimental data fits well to a sliding–rebinding kinetic scheme for X-dimer catch bond formation [18] , [19] . X-ray crystallography, nuclear magnetic resonance (NMR), single-molecule fluorescence resonance energy transfer and live cell experiments suggest that X-dimers serve as kinetic intermediates in the pathway to strand-swap dimer formation and dissociation [6] , [9] , [56] , [57] . However, recent data suggest that cadherin signalling can also be triggered via conformational changes at the X-dimer interface [58] . It is therefore possible that catch bonds serve to strengthen X-dimer linkages and permit the transmission of EC forces to the cell interior in order to facilitate cadherin mediated mechano-transduction. X-dimer catch bonds could also tune the mechanical properties of adhesion junctions by enabling cells to grip strongly under load and lock in place when pulled. MD and SMD Simulation MD and SMD simulations were performed on Amazon Elastic Compute Cloud (Amazon EC2), a resizable cloud computing web service. The crystal structure of the EC1-2 domains of W2A mutants (PDB ID: 3LNH) was used in the simulations. The four missing amino acids at the N-terminal of the EC1 domains were manually added using SWISS-PDBViewer. Simulations were performed with GROMACS 4.5 using GROMOS 53a6 force-field and SPC216 water model. For MD simulations, the X-dimer was placed at the centre of a 11 × 9 × 8 nm 3 tri-clinic box filled with simple point-charge water molecules such that no atom of the protein was closer than 1 nm from the walls of the box. The MD equilibration system consisted at an average of 66,875 atoms. Global charge neutrality of the system was maintained by adding Na + counter-ions to the box as needed. When Ca 2+ ions were eliminated from the EC1-2 linker, they were replaced with Na + ions to provide electro-neutrality. To ensure that the solvated X-dimers have no steric clashes or inappropriate geometries, we first energy minimized the system. Periodic boundary conditions were assumed in all simulations. A cutoff of 1 nm was used for van der Waals interactions. Electrostatic interactions were calculated with a particle mesh technique for Ewald summations with a 1-nm cutoff. We equilibrated the water molecules and ions around the X-dimer in two phases. In the canonical (NVT) phase, the system was established at a constant reference temperature of 300 K using a modified Berendsen thermostat. The pressure of the system was then stabilized under isothermal–isobaric (NPT) conditions using a Parrinello–Rahman barostat. Following equilibration, 10–30 ns MD simulations were run at 2 fs integration steps with Linear Constraint Solver (LINCS); and frames were recorded at 1 ps intervals. We began SMD simulations using the last trajectory of the production MD run as the initial structure. This structure was embedded at the centre of a 12 × 40 × 8 nm 3 tri-clinic box; the system consisted of ~382,340 atoms. The SMD simulations used an umbrella pulling method, that is, a harmonic potential with stiffness k =332 pN nm −1 was applied between the atoms on the C-terminal residue on opposing EC2 domains; while one C α atom served as reference group, the other one was the pulling group. The pulling force was measured at every 2 fs time step ( Supplementary Fig. 8 ). Two constant velocity simulations were carried out, one with a faster pulling rate of 2 nm ns −1 and another at slower velocity of 0.4 nm ns −1 , at 2 fs integration steps with LINCS constraints and frames were recorded every 1 ps. For each SMD simulation, the total number of H-bonds is plotted as a function of time in Supplementary Fig. 9 . MD and SMD structural analysis Structural analysis of X-dimers after MD and SMD simulations were performed using GROMACS 4.5 and VMD 1.9.1. The RMSD in every frame of the MD simulation was calculated using least squares fitting to the initial structure (complete fit with rotation and translation of all atoms). RMSF of all amino acids in the X-dimer were obtained by taking the position of the residues (averaged over the entire simulation) after least squares superposition to the initial structure. The angle between the EC1 and EC2 domains were determined in two steps. We first determined the vector corresponding to the long axis of each domain at every 1 ps interval using VMD. We then calculated the angle between these vectors as a function of time using MATLAB. The calculated angles were compared with the EC1–EC2 angle measured from the original crystal structure that served as the reference. E-cadherin constructs Engineering, purification and biotinylation of W2A cadherin X-dimers have been recently described elsewhere [12] . Briefly, X-dimers fused at the C-terminal to an AviTag (for biotinylation) followed by a His tag were purified from HEK293T cell-conditioned medium. The X-dimers were first purified using Nickel NTA resin (Invitrogen) and subsequently purified using a Superdex200 10/300 GL column (GE Healthcare). After protein purification, the AviTag sequence on the E-cadherin/ATH was biotinylated by using BirA enzyme (BirA500 kit; Avidity). Single-molecule force-clamp measurements Biotinylated cadherin mutants were immobilized on glass coverslips and AFM cantilevers (Olympus, Model: TR400PSA) using methods described previously [29] . Briefly, the cantilevers and coverslips were cleaned and functionalized with amine groups using a 2% v/v solution of 3-aminopropyltriethoxysilane (Sigma) dissolved in acetone. The silanized cantilevers and coverslips were then functionalized with PEG 5000 (Laysan Bio) containing an amine-reactive N -hydroxysuccinimide ester at one end. Seven percent of the PEG spacers presented biotin molecules at their other end. The biotins were first incubated with Streptavidin (Sigma) (0.1 mg ml −1 for 30 min) and then with biotinylated W2A cadherins (60 μg ml −1 for 45 min). Following cadherin immobilization, free binding sites on streptavidin were blocked using a 10-μM solution of biotin. Before beginning an experiment, the functionalized coverslips and AFM tips were incubated in 0.1 mg ml −1 BSA for ~12 h to minimize nonspecific protein binding. An Agilent 5500 AFM with a closed-loop piezoelectric scanner was used in the single-molecule force-clamp experiments. Spring constants of the AFM cantilevers were measured with the thermal fluctuation method [59] ; the cantilevers typically had a spring constant of 0.005 N m −1 . Forces were measured in a pH 7.5 buffer (10 mM Tris, 100 mM NaCl and 10 mM KCl) at different concentrations of CaCl 2 . W2A cadherin mutants, immobilized on the AFM tip and substrate, were allowed to interact for 0.3 s to form X-dimers. The tip was then separated from the surface at a ramp rate of 100 to 700 pN s −1 (data acquisition rate of 12.5 kHz), clamped at a constant force (data acquisition rate of 1 kHz) and bond lifetimes were measured. Each force-clamp measurement was simultaneously converted into a force versus distance trace by measuring the displacement of the piezoelectric stack holding the AFM cantilever. The unbinding distance in every trace was compared with the polymer extension calculated using an extended freely jointed chain model; the model accounted for the non-planar, suprastructure that PEG adopts in water [35] . Since the AFM tip, in our experiments, was pressed gently against the sample to prevent protein denaturation (the maximum force never exceeded 100 pN), there was a systematic error in determining the ‘point of origin’ (POO) of the force–displacement curve (that is, 0 nm). We corrected this systematic error by comparing the POO for every measurement with the POO for force curves where the same AFM probe was pressed against the same surface with nN forces such that cantilever deflection was coupled linearly with piezo displacement [60] . How to cite this article : Manibog, K. et al . Resolving the molecular mechanism of cadherin catch bond formation. Nat. Commun. 5:3941 doi: 10.1038/ncomms4941 (2014).